Tunable ferroelectric polarization and its interplay with spin–orbit coupling in tin iodide perovskites Ferroelectricity is a potentially crucial issue in halide perovskites, breakthrough materials in photovoltaic research. Using density functional theory simulations and symmetry analysis, we show that the lead-free perovskite iodide (FA)SnI 3 , containing the planar formamidinium cation FA, (NH 2 CHNH 2 ) + , is ferroelectric. In fact, the perpendicular arrangement of FA planes, leading to a ‘weak’ polarization, is energetically more stable than parallel arrangements of FA planes, being either antiferroelectric or ‘strong’ ferroelectric. Moreover, we show that the ‘weak’ and ‘strong’ ferroelectric states with the polar axis along different crystallographic directions are energetically competing. Therefore, at least at low temperatures, an electric field could stabilize different states with the polarization rotated by π /4, resulting in a highly tunable ferroelectricity appealing for multistate logic. Intriguingly, the relatively strong spin–orbit coupling in noncentrosymmetric (FA)SnI 3 gives rise to a co-existence of Rashba and Dresselhaus effects and to a spin texture that can be induced, tuned and switched by an electric field controlling the ferroelectric state. One way to meet the growing energy demand of society, is the direct conversion of sunlight into electric power using photovoltaic cells. Increasing the efficiency of solar cells and relying on nontoxic abundant elements are absolutely vital to widely replace other means of energy production. Remarkably, in ferroelectric (FE) photovoltaic devices, where a homogeneous FE material acts as a light-absorbing layer, the electric field can help to separate electron–hole pairs, increasing the photocurrent [1] , [2] . Shift current has been proven to be a main mechanism of the bulk photovoltaic effect in FE oxides [3] , [4] . Research interest in FE photovoltaic cells has been rekindled by the report that the lead iodide perovskite, (MA)PbI 3 , where MA refers to the methylammonium cation (CH 3 NH 3 ) + , possesses ultrafast carrier mobility with a solar-energy-conversion efficiency of the order of 20% (ref. 5 ). In the class of organic/inorganic iodide perovskites (some of them remarkably crystallizing in a polar space group at room temperature) [6] , (MA)PbI 3 has so far been the most promising material, because of a high absorption coefficient for the portion of the electromagnetic spectrum that passes through the atmosphere, combined with relatively long carrier lifetimes [7] . Mitzi et al. [8] , [9] investigated the properties of layered organic–inorganic halides as thin-film transistors and light-emitting diodes. Photovoltaic properties were initially reported by Miyasaka and co-workers for the lead-based perosvkite [10] reporting an efficiency ~2–4%, which subsequently increased to 6.5% (ref. 11 ). Later, it was observed that ‘meso-superstructured solar cells’ [12] result in even higher efficiency [13] . Recent experimental work [14] , [15] , [16] has further improved the efficiency reaching now 17.9% (refs 7 , 17 ). Interestingly, these solar cells show many unusual characteristics, for instance, an anomalous hysteresis in the current–voltage curves [18] that was tentatively related to their FE properties [18] . A full understanding of the hysteresis in (MA)PbI 3 is essential for further progress and is likely to lead to performance improvements [18] , [19] . However, green energy requirements pose serious constraints on the use of Pb-based materials, thus raising the question whether Pb could be replaced by nontoxic elements, such as Sn (refs 20 , 21 , 22 ). Intriguingly, owing to the presence of relatively heavy elements in halide perovskites, spin–orbit coupling (SOC), joint with the noncentrosymmetry of FE materials, might give rise to exotic spin-splitting phenomena [23] , such as Rashba or Dresselhaus effects [24] , [25] , [26] occurring in the relativistic electronic structure of (nonmagnetic) semiconductors. While the Dresselhaus effect was originally formulated for three-dimensional (3D) solids as arising from bulk inversion asymmetry, whereas the Rashba effect was thought to derive from two-dimensional (2D) structural inversion asymmetry, this picture has been recently and nicely revised in an unified perspective [27] , following the discovery of Rashba effects in bulk materials [28] , [29] . Indeed, according to ref. 27 , spin splittings can be classified on the basis of atomic site point groups lacking inversion symmetry, being either nonpolar (Dresselhaus) or polar (Rashba), implying also their possible co-existence. Within this framework, we remark that, despite strong interest in photovoltaic cells based on FE organic/inorganic iodide perovskites, experimental/theoretical studies concerning their FE behaviour and related relativistic effects are very few [2] , [23] , [30] , [31] , [32] , [33] , [34] . The tin iodide (FA)SnI 3 , where FA refers to the formamidinium cation ((NH 2 ) 2 CH) + , is quite unique in that each planar polar cation, FA, can change its dipole direction by rotating around its N···N axis, which is parallel to the crystallographic a axis. Thus, the arrangements of the FA cations in the bc plane determine whether (FA)SnI 3 has a FE or antiferroelectric (anti-FE) structure, and how one FE structure is converted to another one with opposite polarization by coordinated rotations of the FA ions. On the basis of noncollinear-spin density functional theory (DFT) simulations, complemented with a careful symmetry analysis and relativistic GW calculations for the quasiparticle excitation energies, we study minimum energy structures of (FA)SnI 3 . We find that the coordinated rotational motions of the FA cations can lead to a polarization reversal, as well as to a change of the directions of the polar axis, and we examine how the Dresselhaus and Rashba effects arising from SOC and FE polarization depend on the rotational arrangements of the FA cations. We show that, in the minimum energy structure, the plane of every FA cation is perpendicular to those of its surrounding four FA cations, giving rise to a ‘weak’ FE polarization. The ‘strong’ FE and ‘anti’ FE arrangements of the FA cations represent transition states on the pathway between two minimum energy structures with opposite polarization. By examining strong and weak FE arrangement of FA cations with the polar axis oriented in different directions, we show that these states have competing total energy. Our results for (FA)SnI 3 open, therefore, the way to a highly tunable polarization and to a co-existence of electrically tunable ‘bulk’ Dresselhaus and Rashba effects. Structural and FE properties We start by considering the experimental structure of (FA)SnI 3 with space group Amm 2 (ref. 6 ; see strong FE structure in Fig. 1b ). The FA cation is planar and polar with its dipole moment parallel to the C–H bond, as shown in Fig. 1a . The organic cations show a strong FE arrangement with all N···N axes parallel to the a axis, and the dipole pointing into the c direction. The iodine anions of the SnI 3 framework are divided into axial and equatorial ( I ax and I eq , respectively). Here the Sn- I ax -Sn and Sn- I eq -Sn bridges are parallel and perpendicular to the N...N axis of the FA cations. To evaluate the FE polarization from first principles, it is necessary to establish a centrosymmetric reference structure, which is converted to the noncentro-symmetric structures by applying a symmetry-breaking structural distortion. As reference structure, we adopt the anti-FE structure shown in Fig. 1b , in which two FA cations (referred as (I) and (II) in Fig. 1b ) have an anti-FE arrangement along the b axis. In our search for the anti-FE→strong FE interconversion pathway, we considered out-of-phase rotations, where the FA cations on one column undergo a clockwise rotation, whereas those on the neighbouring column undergo a counterclockwise rotation around their N···N axes, as schematically depicted in Fig. 1b . Our DFT calculations show that the theoretical minimum energy structure is not the experimentally reported FE structure [6] . Instead, our lowest energy structure corresponds to an arrangement of the molecules resulting in the weak FE structure shown in Fig. 1b , where the C–H bonds are aligned along the face diagonal, and the C–H bonds in adjacent molecules are rotated by 90° with respect to each other. The anti-FE structure, as well as the experimentally reported strong FE structure [6] , represent transition states for the pathway that converts one minimum energy structure to another one with opposite polarization. 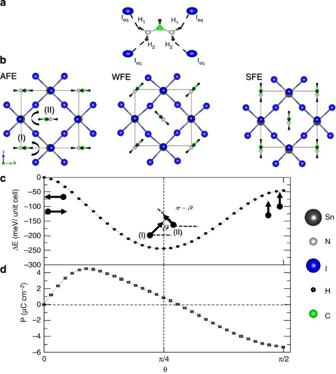Figure 1: Energy and ferroelectric polarization of (FA)SnI3as a function of the FA cation arrangement. The internal atomic positions have been optimized, while the the volume and shape of the unit cell are fixed. (a) Details of thecation making N-H···Ieqcontacts; by symmetry, the molecular dipole moment is directed along the C–H bond. (b) The anti-FE (AFE), weak FE (WFE) and strong FE (SFE) structures as projected into thebcplane. (I) and (II) refer to the two FA cations in the unit cell; the curved arrows denote the rotations of the FA cations around theaaxis. (c) The total energy profile as a function ofθ, taking the anti-FE as reference configuration. In the inset we show the relative orientation of the molecular dipole. (d) The polarization as function ofθwithcas the polar axis. These transition states are ~100 meV per formula-unit higher in energy than the low-energy weak FE structure (see Supplementary Note 1 and Supplementary Figure 1 for further structural details). Figure 1: Energy and ferroelectric polarization of (FA)SnI 3 as a function of the FA cation arrangement. The internal atomic positions have been optimized, while the the volume and shape of the unit cell are fixed. ( a ) Details of the cation making N-H··· I eq contacts; by symmetry, the molecular dipole moment is directed along the C–H bond. ( b ) The anti-FE (AFE), weak FE (WFE) and strong FE (SFE) structures as projected into the bc plane. (I) and (II) refer to the two FA cations in the unit cell; the curved arrows denote the rotations of the FA cations around the a axis. ( c ) The total energy profile as a function of θ , taking the anti-FE as reference configuration. In the inset we show the relative orientation of the molecular dipole. ( d ) The polarization as function of θ with c as the polar axis. Full size image Analysis of the FE polarization The anti-FE structure has a centric space group Pmma , with no net polarization. The weak FE and strong FE structures are described by acentric space groups Pmc 2 1 and Amm 2, respectively, and both display a net FE polarization. In the following, we consider the total polarization, that is, the sum of ionic and electronic contributions. We consider the path from the anti-FE to strong FE structures passing through the weak FE structure by introducing an angle θ . This angle specifies the direction of the C–H bond, whereas the N···N axis is always roughly parallel to the a axis (see Fig. 1b,c ). For θ =0, π /4 and π /2, we obtain the anti-FE, weak FE and strong FE structures, respectively. With this choice, the polarization is always parallel to the c axis, and since all structures possess a band gap, the change of the polarization along the pathway can be calculated using the Berry-phase approach [35] . The two end points (anti-FE and strong FE) are kept fixed, whereas the internal coordinates of all other structures are fully optimized using the nudged elastic band method [36] . 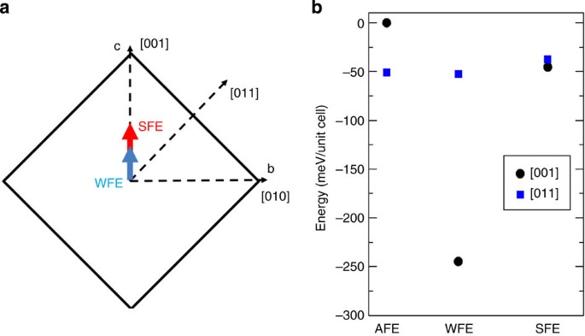Figure 2: Directions of weak FE and strong FE polarizations in (FA)SnI3and dependence of its energy on the dipole orientation of FA. (a) Schematic top view of thebcplane showing the relevant polar directions for strong FE and weak FE arrangements. (b) Relative energies of the anti-FE, weak FE and strong FE arrangements of the FA cations in (FA)SnI3for the cases when the dipole of each FA cation is fixed along [001] and [011]. This approach allows us to take into account the coupling between the molecular rotations and the distortions of the framework (see Supplementary Note 2 and Supplementary Figure 2 ). The total-energy variation and the total polarization as a function of θ are shown in Fig. 1c,d , respectively. The energy is lowered when θ increases, exhibiting a minimum at the weak FE arrangement. Then, the energy increases again towards the strong FE arrangement, which is slightly more stable than the anti-FE one. The polarization sets out from zero for the anti-FE structure, exhibits a maximum between the anti-FE and weak FE structures and then monotonically decreases towards the strong FE state. The overall polarization vanishes and switches its direction along the pathway: this is a result of the balance between opposite contributions of the local FA dipoles and of the SnI 3 framework, as further detailed in the Supplementary Note 2 and Supplementary Figure 2 . The calculated polarization at the DFT level is P weak−FE =0.88 μC cm −2 and P strong−FE =−5.35 μC cm −2 for the weak FE and strong FE structures, respectively. We caution the reader that we limited our study to the smallest unit cell compatible with an antiferroelectric reference structure. Lower energy structures may be possible when using, for example, larger unit cells. However, this goes beyond the present study, since our aim is to highlight the band-structure features due to the interplay between ferroelectricity and SOC and, for this purpose, the smallest unit cell is the most reasonable system to study. We also remark that other polar arrangements for the molecular dipole moments in the pseudocubic structure are possible. If the b and c lattice parameters are equal, which is roughly observed experimentally, states with polarization parallel to these two directions are symmetry equivalent. However, we can also choose to align the C–H bond in the anti-FE and strong FE structure along the ( b + c ) direction (that is, [011]) instead of the b ([010]) or c ([001]) axis. Then, the dipole moment is also parallel to [011] in the strong FE structure. Analogously, it is possible to have weak FE states with polar axis along the [011] direction. The calculated energy variations are shown in Fig. 2b . It is evident that for polarizations along [011] the energy variations between the anti-FE, weak FE and strong FE structures are negligible, and that the weak FE structure with polarization along [001] is lower in energy than any of the other structures. Our analysis of the structures shows that short N-H··· I eq and N-H··· I eq distances occur only for the weak FE structure with the dipole moments parallel to the b or c axis (compare Fig. 1b and Supplementary Note 1 and 2 ). 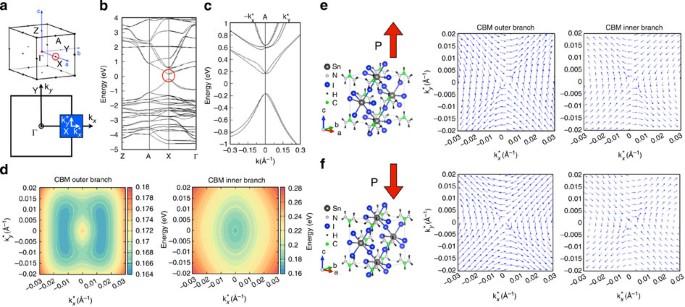Figure 3: Dresselhaus-like spin texture in the conduction band of (FA)SnI3for the strong FE arrangement of the FA cations with their dipoles fixed along [001]. (a) Brillouin zones highlighting the high-symmetry points (top) and the plane orthogonal to the polar axis around the X point (bottom). (b,c) DFT band dispersion relations along the whole Brillouin zone and around the X point. The GW bands are given in theSupplementary Note 6andSupplementary Figure 5. (d) DFT energy profiles for the CBM outer (left) and inner (right) branches of the Rashba—Dresselhaus spin split bands. (e,f) Relative DFT spin textures as a function of the ferroelectric polarization. (e) P-up and outer branch (left), P-up and inner branch (right). (f) P-down and outer branch (left), P-down and outer branch (right). An analysis of the hydrogen bond lengths for the different structures are given in Supplementary Note 3 (see also Supplementary Figure 3, 4 and Supplementary Table I ). Thus, the stability of the weak FE structures is driven by N-H··· I eq hydrogen bonds. Since the latter interactions are weak, it is expected that the polarization orientation can be readily rotated from one direction to another by, for example, applying an external electric field, thus putting forward (FA)SnI 3 as a highly tunable FE . Finally, a comment is in order. Halide perovskites at finite temperatures are likely to exhibit disorder in the molecular orientation due to the associated configurational entropy. Hence, these materials are likely to be paraelectric at room temperature. Indeed, significant disorder was predicted, for example, for CH 3 NH 3 PbI 3 in ref. 37 from molecular dynamics simulations [37] . Figure 2: Directions of weak FE and strong FE polarizations in (FA)SnI 3 and dependence of its energy on the dipole orientation of FA. ( a ) Schematic top view of the bc plane showing the relevant polar directions for strong FE and weak FE arrangements. ( b ) Relative energies of the anti-FE, weak FE and strong FE arrangements of the FA cations in (FA)SnI 3 for the cases when the dipole of each FA cation is fixed along [001] and [011]. Full size image Co-existence of electrically tunable Dresselhaus and Rashba effects The Brillouin Zone of the strong FE structure of (FA)SnI 3 (with the FA dipole direction fixed along [001]) is presented in Fig. 3a , and the related band dispersion is shown in Fig. 3b , indicating the band gap occurring around the X point, as highlighted by the red circle. By projecting the orbitals onto s and p states at the ions, we can determine the predominant character of each band. The conduction band minimum (CBM) shows predominantly Sn 5 p orbital character, whereas the valence band maximum (VBM) is mainly composed of Sn 5 s and I 5 p states. As clearly visible in Fig. 3c , the valence and conduction bands (otherwise twofold degenerate in the absence of SOC) are spin-split and shifted in the k-space away from the high-symmetry point X in presence of SOC, therefore resulting in the so-called ‘inner’ and ‘outer’ branches. In the case of spin-splitting effects, it is customary [26] to define (i) a ‘momentum offset’ (in the k-space), as the difference between the k-point where the band edge is located (including SOC) and the high-symmetry point (X in our case); (ii) an energy splitting, corresponding to the difference between the energy value of a spin-split band at the high-symmetry point (X) and at the band edge. In our case, the energy splittings at the CBM are greater than those at the VBM, and are ~9.4 and 7.7 meV along the and directions, respectively (the and directions are highlighted in the blue inset of Fig. 3a ). The momentum offsets at the CBM are estimated to be 0.016 Å −1 along and 0.013 Å −1 along , whereas those for the VBM are negligible, thus giving rise to a ‘formally indirect’ band gap. Of possible relevance for photovoltaic applications, we note that the different momentum offsets in the conduction and valence bands can possibly affect the probability of radiative recombination of the photo-induced electrons and holes, due to the absence of a formal direct gap [38] . These considerations remain however at the speculative level, as a quantitative evaluation of radiative and nonradiative recombination rates (with and without SOC) is beyond the scope of the present work. Figure 3: Dresselhaus-like spin texture in the conduction band of (FA)SnI 3 for the strong FE arrangement of the FA cations with their dipoles fixed along [001]. ( a ) Brillouin zones highlighting the high-symmetry points (top) and the plane orthogonal to the polar axis around the X point (bottom). ( b , c ) DFT band dispersion relations along the whole Brillouin zone and around the X point. The GW bands are given in the Supplementary Note 6 and Supplementary Figure 5 . ( d ) DFT energy profiles for the CBM outer (left) and inner (right) branches of the Rashba—Dresselhaus spin split bands. ( e , f ) Relative DFT spin textures as a function of the ferroelectric polarization. ( e ) P-up and outer branch (left), P-up and inner branch (right). ( f ) P-down and outer branch (left), P-down and outer branch (right). Full size image Let us now focus on the spin texture of those bands where spin-splitting effects are larger, that is, the CBM. In the plane identified by the and directions (perpendicular to the FE polarization), the outer branch of the spin-split conduction band shows two symmetric energy minima along the direction, while the inner branch displays a cone shape ( Fig. 3d ). These two split bands present nontrivial and opposite spin textures, with spins orthogonal to the crystal momenta along the and axes, but radial along the directions rotated by π /4 ( Fig. 3e ). Such a spin texture differs significantly from the one recently predicted for β -(MA)PbI 3 , β -(MA)SnI 3 and ortho -(MA)SbBr 3 FE halide perovskites, where spins rotate in a circular way on constant energy contours, according to a Rashba-type spin splitting [23] . This calls for a deeper understanding, which we provide in terms of k · p Hamiltonian modelling. Indeed, the SOC-induced band splitting around the CBM can be understood by inspecting the expression of symmetry-allowed terms in the k · p Hamiltonian around the gap [26] . The expression of the effective Hamiltonian is strictly fixed by symmetry. Since the X point preserves time-reversal symmetry, a Kramers pair is observed at the CBM, which is split by SOC away from X. The doublet is well described in a natural basis according to the total angular momentum J =1/2 (refs 23 , 31 ), transforming as the usual Pauli matrices σ x , σ y and σ z . The general expression of the k · p Hamiltonian can hereafter be inferred by taking into account—besides time reversal—the point-group symmetry at X, which is C 2 v . To first order in k *, the SOC-induced term entering the effective Hamiltonian under the considered symmetries takes the form , where α , β denote material-dependent constants ( Supplementary Note 4 and Supplementary Table II ). These constants are not required to be equal under the C 2 v symmetry, in contrast to the aforementioned case of (MA)PbI 3 , where a C 4 v point symmetry imposes α = β , hence leading to a pure Rashba-like term [23] . The SOC term acquires a more transparent form if the local reference system is rotated by π /4 around (that is, the polar axis); in the rotated system the SOC term is rewritten as , where the first and second terms describe a Rashba and a linear Dresselhaus effects [26] , respectively, with coupling constants α R =( α + β )/2 and α D =( α − β )/2. Such a co-existence of Dresselhaus and Rashba terms has been extensively studied in semiconductor quantum wells with C 2 v point symmetry, as n -type heterostructures such as InAs/Al 0.3 Ga 0.7 Sb single quantum well [39] or GaAs/InGaAs quantum wells [40] . In the plane of and , the band dispersion close to the CBM shows a spin-splitting correction , where , which nicely accounts for the predicted band shapes and the two symmetric energy minima along the direction when | β |>| α |. By fitting the conduction bands along , with this spin-splitting correction, we find that at the CBM the Rashba and Dresselhaus coupling terms are α R =0.003 eVÅ and α D =1.19 eVÅ , respectively (values at the VBM cannot be reliably evaluated due to negligible spin splitting). This shows that a rather large Dresselhaus coupling is present and that the Dresselhaus-like term dominates over the Rashba-like, thus explaining the origin of spin textures in (FA)SnI 3 that strongly resemble pure Dresselhaus-type ones ( Supplementary Note 4,5 and Supplementary Table II ). For an increased accuracy, we estimate, within the GW approximation ( Supplementary Note 6 and Supplementary Figure 5 ), the spin splittings at the CBM to be as large as 14.8 and 10.2 meV along and directions, respectively, at momentum offsets from X of 0.022 and 0.018 Å −1 , respectively. The resulting Rashba/Dresselhaus parameters, estimated within GW, α R =0.08 eVÅ and α D =1.24 eVÅ, are not significantly different from those obtained from bare-DFT, thus reinforcing the quantitative DFT estimates made so far. Interplay between ferroelectricity and SOC Since the bulk Rashba α R and Dresselhaus α D constants strongly depend on the potential gradient and inversion-asymmetric environment of the active ions within the material, in turn giving rise to ferroelectricity, one can anticipate changes in the spin splittings and spin texture depending on both the direction and sense of FE polarization. Indeed, the reversal of the polar axis via the application of an external electric field is expected to lead to a switching of the spin texture, as predicted in theoretical studies for bulk GeTe (refs 29 ) and, later on, for β -(MA)PbI 3 , β -(MA)SnI 3 and ortho -(MA)SbBr 3 FE halide perovskites [23] . In Fig. 3e,f we show that the Dresselhaus-like spin textures at the CBM is indeed reversed when going from − P to + P in the FE structure. Qualitatively, the same behaviour is found for the weak FE arrangement, even though the spin-splitting effects are slightly reduced, consistent with the smaller calculated value of polarization. As for the effect of rotating the polar axis from [001] to [011], the same qualitative picture is expected to hold for spin-splitting effects and switchable spin textures in the plane perpendicular to P . In fact, even though the point-group symmetry at the X point is lowered to C s —consisting of a mirror operation whose plane contains the polar axis (taken parallel to ) and —the effective SOC Hamiltonian in the chosen reference frame takes exactly the same expression found for C 2 v symmetry, underlying a co-existence of Rashba and Dresselhaus terms whose relative strength depends again on material specifics. Remarkably, however, we find that the spin splittings in the VBM are larger than in the CBM, where they are almost negligible, when the polar axis is parallel to [011]. Such a change in the electronic structure can be roughly ascribed to the different response of the SnI 3 framework when the dipole direction of the organic cations is rotated, resulting in different hybridization paths whose interplay with the atomic SOC is ultimately responsible for the observed spin-splitting phenomena. The VBM splitting for the strong FE structure of (FA)SnI 3 in which the FA dipole direction is fixed along [011] is as large as 5.4 m e V (3.4 m e V) along with a momentum offset of 0.008 Å −1 (0.007 Å −1 ); the corresponding estimated Rashba/Dresselhaus parameters are α R =1.10 eVÅ and α D =0.18 eVÅ (as before, values at the CBM cannot be reliably evaluated due to negligible spin splitting), resulting in a Rashba-like spin textures with spins rotating in a circular way on constant energy contours. This is clearly seen in Fig. 4 where we show: (a) the unit cell and the polarization along the [011] as well as the plane perpendicular to it; (b) spin splitting of the bands along the two perpendicular directions to the polarization (note that the spin splitting is larger in the valence than in the conduction bands); (c) spin texture in the plane perpendicular to the polarization, showing the characteristic Rashba-like texture, with typical spin switching between the inner and outer branch. 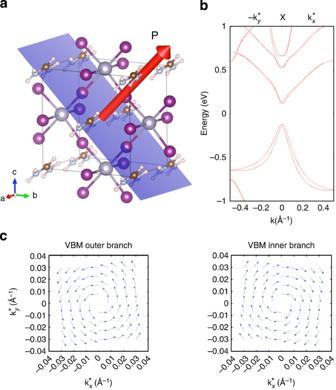Figure 4: Rashba-like spin texture in the valence band of (FA)SnI3for the strong FE arrangement of the FA cations with their dipoles fixed along [011]. (a) Unit cell showing the polarization direction and [011] plane perpendicular to it. (b) Spin spitting in a plane perpendicular to the the direction of the polarization. (c) Characteristic Rashba texture in the plane perpendicular to polarization. Figure 4: Rashba-like spin texture in the valence band of (FA)SnI 3 for the strong FE arrangement of the FA cations with their dipoles fixed along [011]. ( a ) Unit cell showing the polarization direction and [011] plane perpendicular to it. ( b ) Spin spitting in a plane perpendicular to the the direction of the polarization. ( c ) Characteristic Rashba texture in the plane perpendicular to polarization. Full size image Recapitulating this section, our results suggest that spin-splitting effects can be modulated in both the CBM and VBM depending on the polarization direction. When FE polarization is switched from P to − P while keeping the polar axis fixed, the spin textures are found to be fully reversed. On the other hand, the predominance of Dresselhaus and Rashba effects appears to be electrically tunable, as the former (latter) seems to dominate at the CBM (VBM) for polarization along the [001] ([011]) axis. In summary, we have studied a new low-energy structure for (FA)SnI 3 with weak FE order and polarization along the b or c axis. The small-energy barriers between the minimum energy structures and the transition states (namely, strong FE and anti-FE structures) imply that, at least at low temperature, by means of an external electric field, a FE polarization can be induced (from the anti-FE or disordered to the weak FE structure), can be tuned in magnitude (from the weak to the strong FE structure) and in direction (for instance from the [001] to the [011] axis). Therefore, (FA)SnI 3 is expected to exhibit a highly tunable polarization. A sort of similar ‘FE anisotropy’ was previously suggested, by analogy with the magnetic counterpart, in the context of charge-ordered multiferroics [41] ; however, materials that possess that kind of behaviour are very rare, at variance with more common halide perovskites. As the Rashba–Dresselhaus spin texture is tightly linked to the polarization direction, the highly tunable polarization in (FA)SnI 3 opens exciting perspectives in spintronics. The possibility to permanently induce/tune/switch the direction of polarization via an electric field implies a corresponding control over the spin degrees of freedom [23] , [29] . Owing to the high tunability of the FE polarization, the (controllable) co-existence of Rashba and Dresselhaus effects in (FA)SnI 3 can provide new ways to exploit the spin degrees of freedom in photovoltaics. The energy band gap estimated for (FA)SnI 3 based on GW calculations is 1.07 eV, which may be too small for efficient photovoltaic applications. However, one could improve the photovoltaic efficiency, as the electronic properties (in particular, the band gap) can be tuned by a suitable choice of the organic or inorganic components [42] , [43] . Furthermore, the spin texture of (FA)SnI 3 , due to the tunable Rashba–Dresselhaus effects, may give rise to several unique features in the optical properties, such as generating a magnetophotocurrent with possible spin polarization on breaking the time-reversal symmetry of the bulk spin-split bands by applying an external magnetic field [44] , [45] . Since the presence of FE may enhance the photocurrent because of the natural separation of electron and holes [1] , [2] , the tunability of the magnitude and directions of polarization can introduce an additional degree of freedom for collecting the photocurrent, that is, anisotropy of the photocurrent. In this case, one can process the information by electrically writing (for example, stabilizing a given FE state) and optically/electrically reading (for example, detecting a different photocurrent) for a given FE state. Finally, one may envisage the photocurrent being used to extract direct information on the different SOC-induced contributions, such as Rashba and Dresselhaus terms, for example, by means of the photogalvanic effect [39] . All these facts could have interesting applications benefiting from the peculiar electronic and photovoltaic properties of the material, thus opening the possibility of development of new optoelectronic devices [19] . Computational approach Our DFT calculations for (FA)SnI 3 were carried out using the projector-augmented wave method implemented in VASP using the PBEsol functional [46] , [47] , [48] within a noncollinear spin set-up and including SOC. Test calculations have also been performed using the Heyd–Scuseria–Ernzerhof-screened hybrid density functional [49] . We started from the α-phase of (FA)SnI 3 , refined at T =340 K, in the Amm2 space group [6] . The atom positions were optimized until the residual forces were smaller than 0.001 e V Å −1 with the plane-wave cutoff energy of 500 e V and a 6 × 4 × 4 Monkhorst–Pack grid of k-points. Systematic convergence tests with respect to the energy cutoff and k-point sampling were performed, although not shown here. The FE polarization was calculated using the Berry phase method [35] . The use of different van der Waals functionals [50] did not lead to significant differences, demonstrating that the main results presented here are robust. Intermediate structures between θ =0 and θ = π /2 in the analysis of the FE polarization were relaxed using the nudged elastic band method [36] to prevent the formamidinium molecules in the intermediate configurations from rotating back to the minimum energy configuration. An accurate quasiparticle electronic structure was obtained by using a partially self-consistent G W 0 +SOC procedure [51] , [52] , where we have updated the eigenvalues by iterating the Green’s function G while keeping the screening properties W 0 constant at the DFT level. Three iterations were sufficient to achieved a converged solution. A plane-wave basis with an energy cutoff of 420 eV with ~2,100 empty bands on a Γ-centred 4 × 4 × 4 k -mesh and 128 points on the frequency grid are needed to get a converged band structure. The energy cutoff for the response function was set to 150 e V. We made use of the VASP2WANNIER90 interface to interpolate the band structures to a finer grid [53] , [54] . The search of the centric structure, as well as the symmetry analysis, was performed using the PSEUDO and AMPLIMODES tools on the Bilbao Crystallographic Server [55] , [56] . Figures are plotted using the VESTA package [57] . How to cite this article : Stroppa, A. et al. Tunable ferroelectric polarization and its interplay with spin–orbit coupling in tin iodide perovskites. Nat. Commun. 5:5900 doi: 10.1038/ncomms6900 (2014).